Structural analyses of Ca2+/CaM interaction with NaVchannel C-termini reveal mechanisms of calcium-dependent regulation Ca 2+ regulates voltage-gated Na + (Na V ) channels, and perturbed Ca 2+ regulation of Na V function is associated with epilepsy syndromes, autism and cardiac arrhythmias. Understanding the disease mechanisms, however, has been hindered by a lack of structural information and competing models for how Ca 2+ affects Na V channel function. Here we report the crystal structures of two ternary complexes of a human Na V cytosolic C-terminal domain (CTD), a fibroblast growth factor homologous factor and Ca 2+ /calmodulin (Ca 2+ /CaM). These structures rule out direct binding of Ca 2+ to the Na V CTD and uncover new contacts between CaM and the Na V CTD. Probing these new contacts with biochemical and functional experiments allows us to propose a mechanism by which Ca 2+ could regulate Na V channels. Further, our model provides hints towards understanding the molecular basis of the neurologic disorders and cardiac arrhythmias caused by Na V channel mutations. Voltage-gated Na + (Na V ) channels underlie the rapid upstroke of action potentials. Mammalian Na V channels are pseudotetramers with six-transmembrane segment repeats joined by intracellular linkers and flanked by intracellular N- and C-termini. The four repeats, each of which contains a voltage sensor, assemble to form a central pore. Although recent crystal structures of the tetrameric bacterial Na V channel from Arcobacter butzleri (Na V Ab) provided detail about the pore and voltage sensors [1] , [2] , Na V Ab tetramers lack the intracellular linkers and termini of mammalian Na V channels. Those components are of particular interest because they confer isoform-specific regulatory effects, serve as sites of interaction for critical modulatory proteins and are loci for many disease-causing mutations. The C-terminal domain (CTD) is of special interest because it exerts powerful effects upon channel inactivation [3] and is the interaction site for several auxiliary proteins that modulate channel function, such as calmodulin (CaM) and fibroblast growth factor homologous factors (FHFs), both of which regulate excitability through their CTD interactions [4] , [5] . Moreover, many disease-causing mutations localize to Na V CTDs or their associated proteins. Key examples include mutations in SCN1A and SCN2A (which encode the neuronal channels Na V 1.1 and Na V 1.2, respectively) that lead to various epilepsy syndromes, ataxia and autism [6] , [7] , [8] or in the CTD of Na V 1.5, the cardiac Na V channel encoded by SCN5A , which is a hotspot for mutations causing arrhythmias, cardiomyopathy and sudden infant death syndrome [9] , [10] , [11] , [12] , [13] , [14] . Likewise, mutations in FHFs or CaM have been associated with neurodegenerative disorders, cognitive deficits and arrhythmias [14] , [15] , [16] . Structural information about Na V CTDs, however, has been limited. How the associated regulatory proteins influence channel function and how mutations in the CTDs or associated auxiliary proteins perturb channel function and at the molecular level are not well understood. Among the proteins associated with Na V CTDs, CaM is of particular interest because it acts as a sensor for Ca 2+ , which serves as a critical signal of electrical activity, providing powerful feedback regulation upon Na V channel function [17] . Still, how Ca 2+ and CaM affect Na V channels have been controversial since sequence analysis of Na V channels first revealed the presence of potential CaM-binding sites, including an ‘IQ’ motif [5] and a potential Ca 2+ -binding site within the CTD [18] . Obtaining an understanding for CaM regulation of Na V channels has been further complicated by apparent isoform-specific regulation. For example, CaM affects inactivation properties of the neuronal Na V 1.6 but not the skeletal muscle Na V 1.4 (ref. 19 ). For the cardiac Na V 1.5, CaM affects several different properties, including channel inactivation and persistent current [20] , [21] . Nevertheless, the identification of disease-causing mutations within or near the Na V IQ motifs of several Na V isoforms [6] , [20] , [22] , [23] , [24] highlight important roles for CaM. The potential significance of CaM-binding to Na V channels has been further spotlighted by recent exome-sequencing studies in which searches for repeated rare variants or de novo mutations associated with autism identified SCN1A and SCN2A among the small list of loci [25] , [26] , [27] ; several of these catalogued Na V mutations cluster in and around the IQ motif. A major barrier to understand how Ca 2+ and CaM act on Na V channels has been that structural information is limited to Ca 2+ -free CaM (apoCaM) interacting with the CTD. While such studies defined an interaction between the decalcified C-lobe of CaM and the IQ motif [28] , [29] , [30] , those structures were unable to reveal how Ca 2+ affects Na V function and did not provide insight into mechanisms for IQ motif disease mutations, including a familial autism mutation in the neuronal Na V 1.2 channel [7] and a cardiac arrhythmia mutation in the cardiac Na V 1.5 (ref. 20 ) that fall outside of the apoCaM contact sites. Here we present crystal structures of Na V 1.2 and Na V 1.5 CTDs bound to Ca 2+ /CaM. Comparison with our previous structure obtained with apoCaM reveals novel and unexpected Ca 2+ /CaM contacts and stark differences in the overall conformation of the ternary complex, including a Ca 2+ -dependent interaction between the CaM N-lobe and an extended helix that contains the IQ motif. Together, these findings provide a basis for understanding the effects of specific disease-causing mutations within Na V CTD domains. Ternary complex structures of a Na V CTD and FHF and Ca 2+ /CaM To define how Ca 2+ regulates Na V channels, we solved crystal structures of complexes containing a Na V CTD, Ca 2+ /CaM and a FHF. FHFs are constitutive Na V subunits in the brain [4] , [31] and heart [32] and their inclusion allows us to compare Ca 2+ /CaM structures with our previous complex containing apoCaM [30] . We tested several different combinations of FHFs and Na V CTDs with Ca 2+ /CaM and eventually succeeded in crystallizing two ternary complexes: a 6xHis-tagged human Na V 1.5 CTD (amino acids 1,773–1,940), human FGF12B and CaM; and a 6xHis-tagged human Na V 1.2 CTD (amino acids 1,777–1,937), human FGF13U and CaM. The sequences of the Na V CTDs are highly conserved among the subtypes (76% identities between Na V 1.5 and Na V 1.2, and 91% of the amino acids are conserved; Fig. 1a ) and the solution structures of the proximal Na V 1.2 CTD and Na V 1.5 CTD are nearly identical [33] , [34] . Likewise, FGF12B and FGF13U are highly conserved (69% identities), and their crystal structures in the absence of any binding partners are similar [35] . Thus, we anticipated significant similarities between the Na V 1.2- and Na V 1.5-containing complexes. 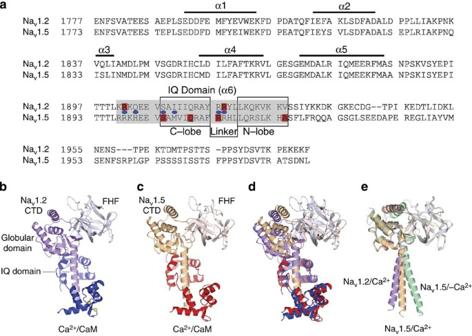Figure 1: Overall architecture of the ternary complexes containing a NaVCTD, CaM and a FHF. (a) Sequence alignment of the NaV1.2 and NaV1.5 CTDs, with structural motifs and the IQ domain indicated. The interaction sites for the CaM N- and C-lobes and the CaM interlobular linker are also indicated. Human disease mutations in NaV1.2 and NaV1.5 clustering in the IQ domain are indicated in red; in blue are the homologous positions of disease mutations in NaV1.1. (b) The NaV1.2/Ca2+structure containing the NaV1.2 CTD (purple), FGF13 (silver) and CaM (blue). (c) The NaV1.5/Ca2+structure containing the NaV1.5 CTD (orange), FGF12 (pink) and CaM (red). (d) Overlay of the NaV1.2/Ca2+and the NaV1.5/Ca2+structures aligned to the IQ motifs. (e) Overlay of the NaV1.2/Ca2+structure; the NaV1.5/Ca2+structure; and the NaV1.5/-Ca2+structure (Protein Data Bank accession code 4DCK), all aligned to the globular domain of the respective CTDs. For clarity, their respective CaM structures were omitted. This arrangement emphasizes the different angles between the globular domains and the IQ motifs among the three structures. Figure 1: Overall architecture of the ternary complexes containing a Na V CTD, CaM and a FHF. ( a ) Sequence alignment of the Na V 1.2 and Na V 1.5 CTDs, with structural motifs and the IQ domain indicated. The interaction sites for the CaM N- and C-lobes and the CaM interlobular linker are also indicated. Human disease mutations in Na V 1.2 and Na V 1.5 clustering in the IQ domain are indicated in red; in blue are the homologous positions of disease mutations in Na V 1.1. ( b ) The Na V 1.2/Ca 2+ structure containing the Na V 1.2 CTD (purple), FGF13 (silver) and CaM (blue). ( c ) The Na V 1.5/Ca 2+ structure containing the Na V 1.5 CTD (orange), FGF12 (pink) and CaM (red). ( d ) Overlay of the Na V 1.2/Ca 2+ and the Na V 1.5/Ca 2+ structures aligned to the IQ motifs. ( e ) Overlay of the Na V 1.2/Ca 2+ structure; the Na V 1.5/Ca 2+ structure; and the Na V 1.5/-Ca 2+ structure (Protein Data Bank accession code 4DCK), all aligned to the globular domain of the respective CTDs. For clarity, their respective CaM structures were omitted. This arrangement emphasizes the different angles between the globular domains and the IQ motifs among the three structures. Full size image Both complexes were expressed in Escherichia coli and purified in the presence of 2 mM Ca 2+ by Co 2+ affinity chromatography followed by size exclusion chromatography. The two ternary complexes (combined M w ~60 kDa) were stable and each eluted in a single peak on a size exclusion column ( Supplementary Fig. 1 ). Their individual profiles were highly similar to each other and to what we observed for the ternary complex containing the Na V 1.5 CTD, FGF13U and CaM purified in EGTA, for which we had demonstrated a stoichiometry of 1:1:1 (ref. 30 ). The complex containing Na V 1.2 CTD, FGF13U and CaM (hereafter referred to as Na V 1.2/Ca 2+ ) was crystallized in the C2 space group with two copies of the ternary complex in each asymmetric unit. The crystals were grown in the presence of 2 mM Ca 2+ and diffracted to 3.02 Å Bragg spacings. The experimental phases were derived by single anomalous dispersion from selenomethionine (SeMet)-substituted crystals and improved by twofold non-crystallographic averaging, which yielded a good-quality electron density map ( Supplementary Fig. 2A ). The final model contains the Na V 1.2 amino acids 1,788–1,929, FGF13U amino acids 11–158 and the CaM amino acids 7–149. The model was refined to R work / R free of 21.5/24.6% ( Table 1 ). The ternary complex containing Na V 1.5 CTD, FGF12B and CaM (hereafter referred to as Na V 1.5/Ca 2+ ) was crystallized in the P3 1 21 space group with one copy of the ternary complex in each asymmetric unit. The crystals were grown in the presence of 2 mM Ca 2+ and diffracted anisotropically to 3.8/5.4/6.0 Å Bragg spacings. Molecular replacement was performed to obtain the phases (see Methods for the details). The final model contains the Na V 1.5 amino acids 1,786–1,927; FGF12B amino acids 12–152; and the CaM amino acids 7–148. Despite the resolution limit, the model refined to good statistics ( R work / R free of 26.2/31.8%) and good geometry ( Table 1 and Methods for the refinement). 2Fo–Fc OMIT map shows a good-quality electron density, supporting the accuracy of the model given the resolution ( Supplementary Fig. 2B ). There is no significant difference in the refinement statistics when the data were truncated to 6.0 Å ( Table 1 ). Table 1 Data collection, phasing and refinement statistics. Full size table Figure 1b,c shows the overall architecture of the Na V 1.2/Ca 2+ and Na V 1.5/Ca 2+ ternary complexes, respectively. In both complexes, the Na V CTD comprises one globular domain that contains an EF-hand fold followed by an extended helix that contains the IQ motif. We refer to this helix as the IQ domain. The FHF binds to the CTD globular domain and CaM binds to the IQ domain. When the Na V 1.5/Ca 2+ and the Na V 1.2/Ca 2+ structures were superimposed with respect to their IQ domain, structural conservation was observed within the region containing the IQ domain and CaM (r.m.s.d. of 1.7 Å; Fig. 1d ). When the two structures (stripped of their respective CaM molecules) are superimposed relative to their respective CTD’s globular domains together with FHFs, both Na V CTD globular domains and FHFs are very similar to the r.m.s.d of 0.89 Å, with their IQ domains out of register ( Fig. 1e ) because of different angles between their CTD’s globular domain (along with FHFs) and their IQ domain. The different angle may reflect an isoform-specific structural difference or inherent flexibility between the two domains of Na V CTD. To focus on the Ca 2+ -dependent conformational changes, we also superimposed our previously solved structure of a ternary complex of Na V 1.5 CTD, FGF13 and CaM crystallized in the absence of Ca 2+ (ref. 30 ), hereafter referred to as Na V 1.5/-Ca 2+ . With the CaM molecules stripped for clarity, Fig. 1e shows that the difference in angle between the respective Na V CTD globular domains and the IQ domains is even more pronounced between Na V 1.5/Ca 2+ and Na V 1.5/-Ca 2+ than between Na V 1.2/Ca 2+ and Na V 1.5/Ca 2+ ( Fig. 1e ). Although it is possible that these rigid-body motions between the CTD globular domains and their respective IQ domains are associated with Ca 2+ binding, these motions can also be due to inherent flexibility between these two domains. As the Na V 1.2/Ca 2+ structure provides higher resolution than the Na V 1.5/Ca 2+ structure and the differences are otherwise minimal, subsequent analyses focus only on the Na V 1.2/Ca 2+ structure. A Ca 2+ -dependent CaM N-lobe interaction with the IQ domain The most significant effects of Ca 2+ are the changes in the interactions between CaM and the respective IQ domains as shown in Fig. 2a,b , in which the Na V 1.2/Ca 2+ and Na V 1.5/-Ca 2+ structures are aligned by their IQ domains. The CaM in the Na V 1.5/-Ca 2+ structure adopts an extended conformation with the α-helical interlobular linker between the CaM/N- and C-lobes holding the N-lobe away from the C-lobe that binds to the proximal portion (IQ motif) of the IQ domain. NMR structures of Ca 2+ -free CaM and an isolated IQ domain peptide from either Na V 1.2 or Na V 1.5 also showed an interaction between the CaM C-lobe and the IQ motif, but not the CaM N/lobe and the IQ domain [28] , [29] . In our new Na V 1.2/Ca 2+ structure, in contrast, the α-helical interlobular linker is unwound, thereby allowing the Ca 2+ -bound CaM N-lobe to envelope the distal portion of the IQ domain and provide additional contacts between the linker and the IQ domain and between the CaM N-lobe and the IQ domain that are not present in the absence of Ca 2+ . These new contacts include residues mutated in channelopathies, as discussed below. 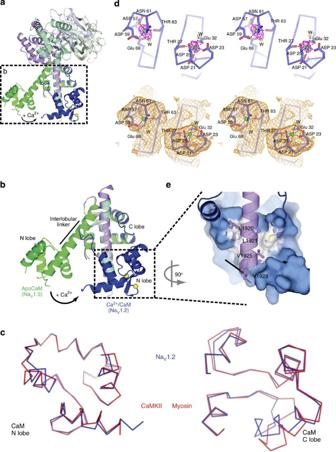Figure 2: Ca2+-dependent calmodulin interactions. (a) Overlay of the NaV1.2/Ca2+and the NaV1.5/-Ca2+structures, both aligned to their IQ domains. Colours for NaV1.2: NaV1.2 CTD (purple), FGF13 (silver) and CaM (blue). Colours for NaV1.5: NaV1.5 CTD (pale green), CaM (dark green), FGF12 (lime). (b) Zoomed-in view of the IQ domains and CaM with the same orientation asa. Ca2+ions are shown as yellow balls. Ca2+-Free-CaM from the NaV1.5/-Ca2+structure is coloured green and Ca2+-CaM from the NaV1.2/Ca2+structure is coloured blue. (c) Cα trace overlay of the Ca2+-loaded CaM N-lobes (left) from the NaV1.2/Ca2+structure (blue); and Ca2+/CaM bound to the CaM-binding peptide in CaMKII (PDB ID 3GP2, red); and the Ca2+-free CaM C-lobes (right) from the NaV1.2/Ca2+structure (blue); and CaM bound to the IQ motif in scallop myosin (PDB ID 2IX7, red). (d) Stereo view of the coordination geometry of the two Ca2+-binding sites in the CaM N-lobe within the NaV1.2/Ca2+structure (top) with the Fo-Fc omit map for Ca2+ions (magenta, 6 σ) and 2Fo–Fc omit map (bottom, salmon, 1 σ). W stands for the water. (e) Zoomed-in view of the CaM/N-lobe (blue) interactions with NaV1.2/Ca2+(purple). Arrow points to Val1928, equivalent to Ala1924 in NaV1.5. Figure 2: Ca 2+ -dependent calmodulin interactions. ( a ) Overlay of the Na V 1.2/Ca 2+ and the Na V 1.5/-Ca 2+ structures, both aligned to their IQ domains. Colours for Na V 1.2: Na V 1.2 CTD (purple), FGF13 (silver) and CaM (blue). Colours for Na V 1.5: Na V 1.5 CTD (pale green), CaM (dark green), FGF12 (lime). ( b ) Zoomed-in view of the IQ domains and CaM with the same orientation as a . Ca 2+ ions are shown as yellow balls. Ca 2+ -Free-CaM from the Na V 1.5/-Ca 2+ structure is coloured green and Ca 2+ -CaM from the Na V 1.2/Ca 2+ structure is coloured blue. ( c ) Cα trace overlay of the Ca 2+ -loaded CaM N-lobes (left) from the Na V 1.2/Ca 2+ structure (blue); and Ca 2+ /CaM bound to the CaM-binding peptide in CaMKII (PDB ID 3GP2, red); and the Ca 2+ -free CaM C-lobes (right) from the Na V 1.2/Ca 2+ structure (blue); and CaM bound to the IQ motif in scallop myosin (PDB ID 2IX7, red). ( d ) Stereo view of the coordination geometry of the two Ca 2+ -binding sites in the CaM N-lobe within the Na V 1.2/Ca 2+ structure (top) with the Fo-Fc omit map for Ca 2+ ions (magenta, 6 σ) and 2Fo–Fc omit map (bottom, salmon, 1 σ). W stands for the water. ( e ) Zoomed-in view of the CaM/N-lobe (blue) interactions with Na V 1.2/Ca 2+ (purple). Arrow points to Val1928, equivalent to Ala1924 in Na V 1.5. Full size image Superposition of Na V 1.5/-Ca 2+ and Na V 1.2/Ca 2+ structures shows that there are only minor conformational changes with respect to the CaM C-lobe. In both structures, the CaM C-lobe adopts the ‘semi-open’ conformation ( Fig. 2c ) that was first described for apoCaM bound to an IQ motif from an unconventional myosin [36] . Significant conformational changes, however, occurred within the N-lobe of CaM, which assumes a ‘closed’ conformation in the Na V 1.2/Ca 2+ structure ( Fig. 2c,d ), similar to the conformation observed for the N-lobe of Ca 2+ /CaM bound to its target peptide in CaMKII [37] . For comparison, in the Na V 1.5/-Ca 2+ structure the unbound CaM N-lobe displays the ‘semi-open’ conformation [30] . In addition, the arrangement of CaM lobes with respect to the IQ domain is novel to the best of our knowledge (see Discussion for further details). These conformation differences of the individual CaM lobes in the Na V 1.2/Ca 2+ structure suggested that the C-lobe was unlikely to be fully occupied, while the N-lobe is saturated with Ca 2+ . To test this hypothesis we collected data for the Na V 1.2/Ca 2+ crystals at a long wavelength (1.55 Å), for which the anomalous scattering power of Ca 2+ (f″~1.2 e) is higher than that of sulphur (~0.6 e), while that of Mg 2+ is nearly silent (~0.1 e). Although we observed strong anomalous difference Fourier peaks in the Ca 2+ -binding loops of the CaM N-lobes, only weak peaks were observed in the Ca 2+ -binding loops of the CaM C-lobe ( Supplementary Fig. 3 ), suggesting that the affinity for Ca 2+ in the CaM C-lobe of Na V 1.2/Ca 2+ is low (compared with the CaM N-lobe) and that the CaM C lobe is only partially occupied with Ca 2+ , consistent with the semi-open conformation of the CaM C-lobe. This newly discovered interaction between the CaM N-lobe and the distal C-terminal portion of the IQ domain is driven mainly through van der Waals forces ( Fig. 2e ), burying Na V 1.2 hydrophobic side chains (Leu1,920, Leu1,921, Val1,925 and Val1,928) and has functional and disease-related implications. First, this additional interaction between the distal IQ domain and the CaM N-lobe offers an explanation for a previous report that an Ala1,924Thr mutation in the cardiac Na V 1.5 channel (equivalent to Val1928 in Na V 1.2) causes the life-threatening arrhythmia Brugada Syndrome and eliminates the Ca 2+ /CaM-dependent slow inactivation observed for the wild-type Na V 1.5 channel [20] . We hypothesized that the Ala1924Thr mutation in the Na V 1.5 CTD affected the affinity for Ca 2+ /CaM and tested the hypothesis by isothermal calorimetry (ITC). Indeed, in the presence of saturating 5 mM Ca 2+ , the mutation reduced the affinity for Ca 2+ /CaM by approximately threefold compared with the wild-type Na V 1.5 CTD ( Supplementary Fig. 4A and Table 2 ). In contrast, the affinity of the mutant Na V 1.5 CTD for CaM in the absence of Ca 2+ was mildly increased ( Table 2 ). Second, we found that the CaM N-lobe interaction with the distal IQ domain provides a significant boost to the affinity of Ca 2+ /CaM for the Na V CTD. A previous report using ITC [38] had found the affinity of Ca 2+ /CaM for a Na V 1.5 peptide containing the IQ motif to be ~2.1 μM. Those thermodynamic parameters, however, were obtained in experiments employing an IQ domain in which the newly discovered CaM N-lobe contact site is truncated. We therefore performed ITC with a longer Na V 1.5 CTD (through amino acid 1,940) and observed a significantly higher affinity for both Ca 2+ /CaM and apoCaM (~100 nM, as shown in Supplementary Fig. 4A,B and Table 2 ). To assure that the lower K d values we obtained were indeed because of the longer CTD and not because of technical differences, we measured the affinity of CaM for the Na V 1.5 CTD truncated at amino acid 1,924, for which we obtained a value of 2.0±0.4 μM in 5 mM Ca 2+ ( Table 2 and Supplementary Fig. 4B ). This result is in excellent agreement with the value previously obtained [38] , thereby allowing us to benchmark our thermodynamic data against that report. Thus, the ~20-fold higher affinity for CaM obtained with the longer CTD highlights critical contributions of the more distal IQ domain residues. Comparison of the N values of interactions for Ca 2+ /CaM with the two CTDs by ITC ( Table 2 ) further demonstrates the importance of the more distal residues in the IQ domain. For the shorter CTD, the N value of the Ca 2+ /CaM–CTD interaction is close to ~0.5 (0.38 in our measurement, and 0.56 previously reported [38] ), suggesting that one Ca 2+ /CaM can bind two CTDs. The N value we obtained for the longer CTD was doubled (0.84), suggesting that one Ca 2+ /CaM binds one CTD, and fits well with our crystallographic observation that both N- and C-lobes simultaneously bind to different sites within the IQ domain of Na V CTD. Consistent with our observation, N value of the interaction between Ca 2+ /CaM and Ala1924Thr of the longer CTD is reduced to half of the wild type (0.42; Table 2 ). Thus, these data underlined the importance of the interaction between CaM and the more distal region of the IQ domain and supported a model in which there are simultaneous interactions of the two CaM lobes (at different sites on the IQ domain). Table 2 Thermodynamic parameters for CaM interaction with the Na V 1.5 CTD. Full size table Ca 2+ -dependent changes and disease mechanisms While the new CaM N-lobe contact with the Na V 1.2 CTD is the most obvious Ca 2+ -dependent structural change, we also identified additional new Ca 2+ /CaM contact sites within the Na V 1.2 IQ domain, which may provide insight for several other Na V channelopathies. For example, Arg1918 ( Fig. 3a,b ), which contacts Asp79 and Ser82 in the CaM interlobular linker in the Ca 2+ -loaded complex (but not in the apoCaM structure), was reported in a patient with febrile seizures and childhood absence epilepsy [23] , and mutation of the equivalent Arg1928 in the homologous Na V 1.1 was found in a patient with severe myoclonic epilepsy of infancy [24] . 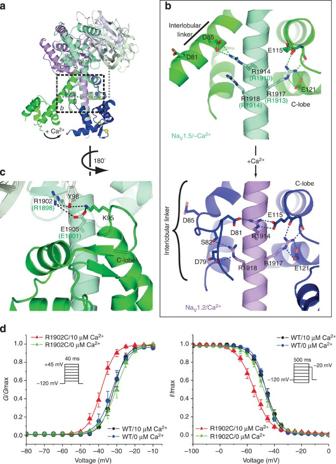Figure 3: Ca2+-dependent structural changes highlight mechanisms for NaVchannel dysfunction with disease mutations. (a) Overall structure of the NaV1.2/Ca2+and NaV1.5/-Ca2+complexes for orientation, as inFig. 2a. Boxed area shows the relative region for focus inb,c. (b) Zoomed view of the NaV1.5/-Ca2+and NaV1.2/Ca2+structures demonstrating the Ca2+-dependent changes in interaction between the NaVCTD and the CaM C-lobe and CaM interlobular linker. For comparison, the labelling for the Arg residues within the NaV1.5 CTD employs the corresponding numbers for NaV1.2; and the NaV1.5 numbers are shown in parentheses. (c) Zoomed view of the NaV1.5/-Ca2+structure focusing on the interaction between Arg 1898 (Arg 1902 in NaV1.2) in the NaV1.5 CTD and Lys 95 in CaM via Glu1901 (Glu1905 in NaV1.2) and Tyr98 in FGF13. As inb, the numbering within the CTD corresponds to the NaV1.2 sequence and the NaV1.5 equivalents are in parentheses. (d) Activation and steady-state inactivation relationships in 0 mM Ca2+or 10 μM-free Ca2+in the recording pipette for wild-type NaV1.2 or the Arg1902Cys CaM N-lobe interaction mutant. Summary data and statistics are provided inTable 1. Figure 3: Ca 2+ -dependent structural changes highlight mechanisms for Na V channel dysfunction with disease mutations. ( a ) Overall structure of the Na V 1.2/Ca 2+ and Na V 1.5/-Ca 2+ complexes for orientation, as in Fig. 2a . Boxed area shows the relative region for focus in b , c . ( b ) Zoomed view of the Na V 1.5/-Ca 2+ and Na V 1.2/Ca 2+ structures demonstrating the Ca 2+ -dependent changes in interaction between the Na V CTD and the CaM C-lobe and CaM interlobular linker. For comparison, the labelling for the Arg residues within the Na V 1.5 CTD employs the corresponding numbers for Na V 1.2; and the Na V 1.5 numbers are shown in parentheses. ( c ) Zoomed view of the Na V 1.5/-Ca 2+ structure focusing on the interaction between Arg 1898 (Arg 1902 in Na V 1.2) in the Na V 1.5 CTD and Lys 95 in CaM via Glu1901 (Glu1905 in Na V 1.2) and Tyr98 in FGF13. As in b , the numbering within the CTD corresponds to the Na V 1.2 sequence and the Na V 1.5 equivalents are in parentheses. ( d ) Activation and steady-state inactivation relationships in 0 mM Ca 2+ or 10 μM-free Ca 2+ in the recording pipette for wild-type Na V 1.2 or the Arg1902Cys CaM N-lobe interaction mutant. Summary data and statistics are provided in Table 1 . Full size image In addition, of particular interest was a familial autism mutation Arg1902Cys in Na V 1.2 (ref. 7 ) especially since recent analyses of rare de novo mutations in subjects with autism have identified SCN2A as one of a handful of high-confidence autism spectrum disorder genes [25] , [39] . Arg1902 sits at the hinge between the CTD globular domain and the IQ domain helix ( Fig. 3c ). We had previously found that the Arg1902Cys mutation conferred a Ca 2+ /CaM-dependent conformational change indicated by a significant Ca 2+ -dependent shift in migration on a size exclusion column of a Na V 1.2 CTD/CaM binary complex that was not observed with the wild-type complex [21] . Although Arg1902 (or the Arg1898 equivalent in Na V 1.5) does not make any direct contacts with CaM either in the presence or in the absence of Ca 2+ , it interacts with the side chain of Glu1905 (Glu1901 in Na V 1.5) one turn below along the IQ domain helix and also forms cation-π interaction with the side chain of Tyr98 in FGF13U in the Na V 1.5/-Ca 2+ structure. Tyr98 in FGF13 and Glu1905 in Na V 1.2 (Glu1901 in Na V 1.5) also interact with Lys95 within the third CaM EF-hand in the CaM C-lobe. Interestingly, Glu1905 in Na V 1.2, Tyr98 in FGF13U and Lys95 in CaM are the only residues within the ternary complex that make interactions with each of the other partners. Thus, we suspected that the relayed interactions from Lys95 (CaM) through Glu1905 (Nav IQ domain) to Arg1902 (Nav globular domain), stabilized by the cation-π interaction with Tyr98 in FGF13, suppress the Ca 2+ -dependence of Na V 1.2 channels and that disruption of these interactions would affect Ca 2+ -dependent regulation of Na V 1.2 channels ( Fig. 3c ). We tested this hypothesis in two ways. First, we expressed either wild-type or Arg1902Cys-mutant Na V 1.2 along with FGF14, the best characterized neuronal FHF [4] , [31] , [40] in HEK293 cells, in which endogenous CaM is abundant, and recorded Na + currents in the presence of saturating internal Ca 2+ or nominally zero internal Ca 2+ ( Supplementary Fig. 5 ) For wild-type Na V 1.2, inclusion of 10 μM Ca 2+ in the patch pipette did not affect peak current density, the V 1/2 of activation or the V 1/2 of steady-state inactivation. In contrast, for the Arg1902Cys mutant the addition of Ca 2+ induced a large approximately −10 mV shift in the V 1/2 of steady-state activation and inactivation ( Fig. 3d , Supplementary Fig. 6A and Supplementary Table 1 ). To test further our hypothesis that disruption of the Na V CTD to CaM relay affected Ca 2+ -dependent regulation of Na V 1.2, we ablated the key intermediary by mutating Na V 1.2 Glu1905 to Gln. Recordings from the Glu1905Gln-mutant channels phenocopied those from the Arg1902Cys-mutant channels ( Supplementary Fig. 6A and Supplementary Table 1 ). Second, to test the proposed role of Arg1902 in the relayed interactions in Na V 1.2 CTD/apoCaM, we measured the affinity of apoCaM for the wild-type and Arg1902Cys-mutant Na V 1.2 CTDs by ITC. Consistent with our hypothesis, the Arg1902Cys mutation reduced affinity of apoCaM for the Na V 1.2 CTD significantly ( Table 3 and Supplementary Fig. 4C ). We did not observe a difference in affinity for Ca 2+ /CaM between the wild-type and the Arg1902Cys-mutant CTD ( Table 3 and Supplementary Fig. 4D ). As our ITC measurement in the presence of Ca 2+ could be complicated by an additional binding process because of Ca 2+ -loading of the CaM C-lobe, which is essentially unoccupied in the Na V 1.2/+Ca 2+ structure ( Supplementary Fig. 3 ), we therefore prepared CaM in which the third and fourth EF hands were mutated to ablate Ca 2+ binding to the CaM C-lobe [41] and repeated the ITC measurements with this crippled CaM 34 mutant. The ITC experiment with the CaM 34 mutant showed a reduced affinity for the Arg1902Cys mutant compared with the wild CTD in the presence of Ca 2+ ( Table 3 and Supplementary Fig. 4E ). Thus, these data are consistent with the previously observed shift in mobility on gel filtration of the Arg1902Cys/CaM binary complex [21] and suggest that by disrupting the relayed interactions to CaM the familial autism Na V 1.2 Arg1902Cys mutation revealed Ca 2+ -dependent effects upon channel function that were suppressed in the wild-type channel. Table 3 Thermodynamic parameters for CaM interaction with the Na V 1.2 CTD. Full size table We next investigated whether the Ca 2+ -dependent interaction of the CaM N-lobe was required for the Ca 2+ -dependent regulation of Na V 1.2 exposed by the Arg1902Cys mutation. We mutated Val1925, one of the Na V 1.2 hydrophobic side chains buried by the calcified CaM N-lobe (see Fig. 2e ), to Lys and examined how this mutant affected the Ca 2+ -dependent shift in activation and steady-state inactivation in the context of the Arg1902Cys mutant. With this additional Val1925Lys mutation, the Arg1902Cys mutant no longer displayed any Ca 2+ -dependent effects on either activation or steady-state inactivation ( Supplementary Fig. 6B and Supplementary Table 1 ), thereby implicating a requirement for the interaction between the calcified CaM N-lobe and Na V 1.2. When analysed independently, Val1925Lys did not expose any Ca 2+ -dependent regulation ( Supplementary Fig. 6B and Supplementary Table 1 ). Ca 2+ binding is restricted to CaM Our analyses suggested that Ca 2+ -dependent regulation of Na V channel function derives from Ca 2+ -dependent changes in the interaction between CaM and the Na V CTD, yet it has previously been suggested that Ca 2+ also affects Na V channels by binding directly to an EF-hand motif within the Na V CTD influences Na V channel function [18] , [34] , [42] . To query whether Ca 2+ can bind directly to the Na V CTD EF-hand motif, we used our anomalous scattering studies. Even though we detected anomalous difference signals from many sulphur atoms (in methionines) whose signal is approximately twofold weaker than that for Ca 2+ , we did not detect anomalous difference signal for Ca 2+ within the proposed Ca 2+ -binding loops ( Fig. 4a ) and we observed a strong signal for Ca 2+ bound to the CaM N-lobe ( Supplementary Fig. 3 ). Comparing the acidic and polar residues proposed to coordinate Ca 2+ in the putative Na V CTD EF-hand [18] with those in the Ca 2+ -binding EF hands in the CaM N-lobe of the associated CaM provides an explanation. While both EF hands of the Ca 2+ -loaded CaM N-lobe contain a sufficient number of acidic and polar residues (a total of five) positioned to coordinate Ca 2+ in an optimal geometry ( Fig. 4b and see Fig. 2d ), the Na V CTD EF hand does not ( Fig. 4b ). Thus, we conclude that the Na V CTD EF hand does not likely bind Ca 2+ ; Ca 2+ -dependent effects on Na V channel function are more likely mediated via CaM. 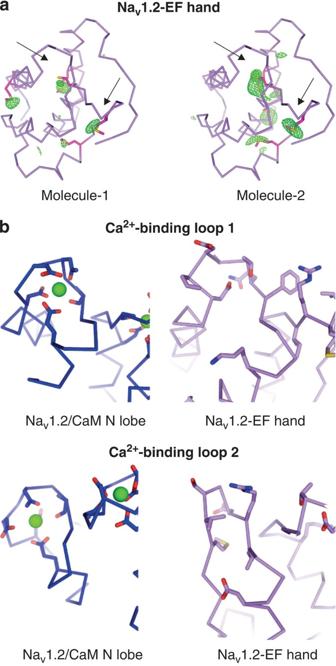Figure 4: The NaVCTD EF hand does not bind Ca2+. (a) Anomalous difference Fourier map for two CaMs in the asymmetric unit from the NaV1.2 CTD crystal. The map was calculated using data from 25.0 to 5.5 Å of the native crystal using the final model phases. The anomalous difference peaks, coloured in green mesh, are contoured at 2.8σThe arrows indicate the expected positions of Ca2+in CaM. Side chains of methionines are shown. (b) Comparison of the first and second Ca2+-binding loop in the CaM/N-lobe with the EF hand motif from the NaV1.2 CTD. Side chains involved in Ca2+coordination in the Ca2+-binding loops of EF hands are shown. Ca2+is shown as a green ball. Figure 4: The Na V CTD EF hand does not bind Ca 2+ . ( a ) Anomalous difference Fourier map for two CaMs in the asymmetric unit from the Na V 1.2 CTD crystal. The map was calculated using data from 25.0 to 5.5 Å of the native crystal using the final model phases. The anomalous difference peaks, coloured in green mesh, are contoured at 2.8 σ The arrows indicate the expected positions of Ca 2+ in CaM. Side chains of methionines are shown. ( b ) Comparison of the first and second Ca 2+ -binding loop in the CaM/N-lobe with the EF hand motif from the Na V 1.2 CTD. Side chains involved in Ca 2+ coordination in the Ca 2+ -binding loops of EF hands are shown. Ca 2+ is shown as a green ball. Full size image Whether and how Ca 2+ contributes to the regulation of voltage-gated Na V currents has been a focus of significant controversy since potential CaM-binding sites were first identified within Na V CTDs [5] . Our new structural model with Ca 2+ /CaM bound to the Na V 1.2 CTD, in context with previous structures demonstrating the interaction of apoCaM with various Na V CTDs [28] , [29] , [30] , reveals novel and unexpected interactions between the Ca 2+ -loaded CaM and the Na V CTD. The apoCaM structures showed that the CaM C-lobe is anchored to the signature IQ motif within the extended IQ domain. On the basis of our new structural, biochemical and functional data, we propose that a major action of Ca 2+ is to induce a conformational switch in the anchored CaM so that the CaM N-lobe swings into contact with the distal IQ domain, while the Ca 2+ -free CaM C-lobe remains anchored to the IQ motif ( Fig. 2b ). Interestingly, the new contact site for the calcified CaM N-lobe sits within a previously identified peptide that, when isolated from the adjacent IQ motif peptide, could only bind Ca 2+ -loaded CaM, in contrast to the IQ motif that supported apoCaM binding over Ca 2+ /CaM binding [5] . In addition, we observed that Ca 2+ induces rearrangements between the Na V CTD and the CaM intralobular linker, and between the Na V CTD and the CaM C-lobe ( Fig. 3b ). We hypothesize that, together, these conformational changes may be propagated to the adjacent domain IV (DIV) transmembrane region of the channel to thereby affect Na V function in an isoform-specific manner. Since our structures do not contain the transmembrane region of the channel, our model cannot explain how the conformational changes propagate to DIV. However, it is known that the conformational change of DIV voltage sensor (S4) is the rate-limiting step for channel inactivation [43] , [44] . Thus, the Na V CTD is in an advantageous position to affect channel gating. Interestingly, the specific Ca 2+ /CaM-dependent effects appear to vary among different Na V channels [19] . Our data add to that concept in which we found that the wild-type Na V 1.2 channel, not previously studied, was insensitive to Ca 2+ /CaM for the parameters we studied at either nominally zero or saturating (~10 μM) intracellular Ca 2+ . While the specific concentrations of internal Ca 2+ studied here are outside the range of physiologic Ca 2+ in neurons, these two levels allowed us to explore the bounds of Ca 2+ , and correlate to our structures, obtained in the absence or presence of Ca 2+ . These functional studies were also performed in the presence of a FHF, which was a component of the crystallized ternary complexes. Whether FHFs influence the Ca 2+ dependence of Na V currents has not yet been analysed. However, their inclusion in the functional studies is appropriate not only because of their presence in the crystal structures but also because of growing evidence that FHFs are important regulators of Na V currents in the neurons and cardiomyocytes [4] , [16] , [32] , [45] in which Na V 1.2 and Na V 1.5 are expressed. Nevertheless, the familial autism mutation Arg1902Cys introduced a large Ca 2+ -dependent shift in both channel activation and steady-state inactivation ( Fig. 3 and discussed below). A gain-of-function effect of a channelopathic mutation is reminiscent to the mechanism by which mutations in Na V 1.5 lead to Long QT Syndrome [9] , [10] and in some Na V 1.2 mutations associated with epilepsy [46] . Combined with analysis of the Na V 1.2/Ca 2+ structure, our functional data suggest that the relayed interactions from Lys95 (CaM) through Glu1905 (Nav IQ domain) to Arg1902 (Nav globular domain) mask a Ca 2+ -dependent shift in wild-type Na V 1.2 that is revealed by the Arg1902Cys familial autism mutant when the relay is disrupted. It is noteworthy that an Asp96Val mutation adjacent to Lys95 in CaM, recently reported in a patient with an arrhythmia syndrome, was also associated with moderate cognitive impairment [14] . Taken together, we suggest that similar Ca 2+ -induced conformational changes of CaM in both Na V 1.2 and Na V 1.5 (interactions of the CaM N-lobe to the distal IQ domain of Na V CTD) might be responsible for Ca 2+ -dependent regulation, and that their functional effects are isoform-specific. The concept that Ca 2+ -dependent regulation may be isoform-specific is consistent with a recent report showing that a rapid increase in intracellular Ca 2+ diminished transient Na V currents through Na V 1.4, but not through the Na V 1.5 isoform [47] . With regard to Na V 1.2, only Arg1902Cys or Glu1905Gln unveiled a Ca 2+ -dependent functional effect. We reasoned that there are possible reasons for these isoform-specific differences of Ca 2+ dependence. First, in the context of the full-length channels, it is possible that the conformational changes at the CTD could propagate to the DIV transmembrane region of the channel differently depending on the isoforms. The apparent isoform-specific difference in the angle between the Na V globular domain and the extended IQ domain reported herein ( Fig. 1e ) provide one possibility. For example, perhaps the difference in the angle within Na V 1.2 masks the Ca 2+ -dependent changes in Na V 1.2 wild-type channel function initiated by the Ca 2+ -dependent CaM N-lobe interaction. Second, it is possible that there are unexamined functional parameters that are more relevant to Ca 2+ -dependent regulations that are less-isoform-specific. Third, it is possible that Ca 2+ /CaM does not mediate the observed Ca 2+ -dependent changes in functions of Na V 1.2 Arg1902Cys or Glu1905Gln. However, the fact that Val1925Lys mutation (in the background of Arg1902Cys) abolishes the Ca 2+ -dependent functional effect eliminates this possibility, as Val1925Lys would disrupt the binding of the CaM N-lobe to the distal IQ motif of Na V 1.2. While mutagenesis studies have yielded suggestions about how Ca 2+ /CaM regulates Na V channel function [18] , [19] , [21] , [38] , [42] , [48] , [49] , human disease mutations can be particularly revealing. By identifying new Ca 2+ /CaM-dependent contacts with the Na V CTD and demonstrating Ca 2+ -dependent conformation changes within the complex, our data provide a context in which to consider the effects of disease mutations that affect Na V CTD–CaM interaction. Several epilepsy mutations in Na V 1.1 or Na V 1.2 are in residues that make different contacts with Ca 2+ /CaM compared with apoCaM ( Fig. 3 ) as are additional Na V 1.1 and Na V 1.2 mutations associated with sporadic and familial cases of autism [7] , [25] , [26] . Further, our analysis of the effects of the Na V 1.2 Arg1902Cys familial autism mutation demonstrates that disruption of the wild-type interaction between the CaM C-lobe and the CTD induces a Ca 2+ -dependent change for the mutant Na V 1.2 channel function. The marked hyperpolarizing shift in both Na V 1.2 activation and inactivation induced by the Arg1902Cys autism mutation would affect neuronal excitability in Na V 1.2-expressing neurons, thus leading to an imbalance between excitation and inhibition known to drive neuropsychiatric phenotypes [50] . In addition, our identification of the Ca 2+ -dependent CaM N-lobe interaction with the distal IQ domain, not predicted by previous structural studies, provides a molecular mechanism for the Ca 2+ -dependent dysfunction of the Na V 1.5 Ala1924Thr Brugada Syndrome mutation [20] . Finally, our data provide a potential mechanism for the recently described mutations in CaM associated with arrhythmias and cognitive deficits [14] . The Ca 2+ -loaded ternary complexes present several unusual and novel features for a CaM-containing complex. Among these are the dissimilar conformations of the CaM N-lobe and CaM C-lobe when calcified CaM is bound to the IQ domain ( Fig. 2c ). While the different conformations of the individual CaM lobes in our structures mirror the CaM lobe conformations seen in the SK K + channel structure, the interactions between CaM and its target peptide(s) are markedly different. Within the SK K + channel homotetramer, the calcified CaM N-lobe wraps around one helix from the C terminus of a protomer but the apoCaM C-lobe interacts with two helices from a different protomer within the tetramer [51] . Split roles for CaM lobes have also been suggested for Ca 2+ -dependent regulation of Ca V channels [52] , [53] , [54] , with one lobe responsible for mediating changes to global Ca 2+ , while the other responds to changes in local Ca 2+ . Comparison of our structures with Ca V Ca 2+ channel-derived structure provides an interesting contrast in structure and mechanisms by which Ca 2+ regulates ion channel function, particularly since voltage-gated Na + channels and Ca 2+ channels are similar in sequence within their proximal CTDs. The similarities include not only the IQ domain to which CaM binds but also an EF hand motif in the Ca V 1.2 L-type Ca 2+ channel that was hypothesized to serve as a site for Ca 2+ -dependent regulation [55] but (similar to the EF hand in the Na V CTD) has also never been shown to bind Ca 2+ with a physiologically meaningful affinity. In spite of these similarities in sequence, structures of the Ca V CTDs bound to CaM are surprisingly different from what we observe for the Na V CTDs. Foremost among these differences is that the Ca V CTD/CaM complexes crystallized as a dimer of CTDs, and each CTD interacted with two CaM molecules for an overall stoichiometry of four CaM and two CTDs [56] , [57] . Whether the dimerization of channels observed in the structure is functionally relevant has been debated. Nevertheless, the 2:1 stoichiometry between CaM and the Ca V 1.2 CTD contrasts markedly with the 1:1 stoichiometry between CaM and a Na V CTD. With these differences, it is not surprising that the overall fold of the Ca V 1.2 CTD does not resemble the Na V CTDs. Even focusing specifically on the interactions between Ca 2+ /CaM and the respective IQ domains, the structures reveal stark differences ( Fig. 5a–c ). First, the arrangement of CaM with respect to the Na V IQ domain is very different than Ca V IQ domains. In both Ca V 1.2 and Ca V 2.1 IQ domains, CaM wraps around the IQ motif in a right-handed helical manner, regardless of the relative orientation of the IQ motifs (parallel or antiparallel to CaM lobes). On the contrary, CaM wraps around the Na V IQ domain in a left-handed helical manner. Second, the overall Ca 2+ /CaM footprint on the Na V IQ domain is longer. The signature IQ motif in Ca V channels forms a central anchor for Ca 2+ /CaM interactions with both CaM lobes, while the IQ motif residues in the Na V structures form contacts mostly with the CaM’s Ca 2+ -free C-lobe. Thus, the Ca 2+ /CaM N-lobe is located further towards the C terminus on the Na V IQ domains compared with the Ca V IQ domains. A search of the Dali database [58] suggesting that the CaM conformation in the Na V 1.2/Ca 2+ and Na V 1.5/Ca 2+ structures is novel. 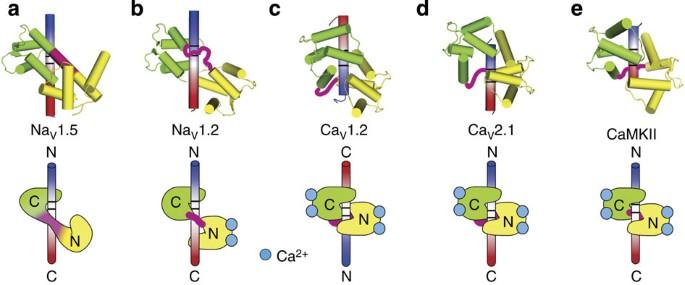Figure 5: CaM conformations when bound to NaVchannels compared with CaVchannels and CaMKII. (a–e) Unique arrangement of CaM relative to the IQ domains in the NaV1.5/-Ca2+structure (a), the NaV1.2/Ca2+structure (b); a CaV1.2 structure (c, PDB ID: 2BE6); a CaV2.1 structure (d, PDB ID: 3DVM) and autoinhibitory (CaM binding) peptide in CaMKII (e, PDB ID: 1CDM). CaM N-lobe and C-lobe are coloured yellow and green, respectively, and the orientation of IQ motifs or autoinhibitory peptide is indicated with a colour gradient (N terminus blue and C terminus red). The positions of IQ(M) amino-acid residues on the IQ domains or the302AI303amino-acid residues in the CaMKII autoinhibitory peptide are demarcated with two black lines. The cartoon figures are shown below each structure to illustrate the difference of the CaM–NaV1.2 interactions. CaM wraps around the NaVIQ domains in the left-handed manner in contrast to the right-handed wrapping seen in CaVstructures and in CaMKII. Figure 5: CaM conformations when bound to Na V channels compared with Ca V channels and CaMKII. ( a–e ) Unique arrangement of CaM relative to the IQ domains in the Na V 1.5/-Ca 2+ structure ( a ), the Na V 1.2/Ca 2+ structure ( b ); a Ca V 1.2 structure ( c , PDB ID: 2BE6); a Ca V 2.1 structure ( d , PDB ID: 3DVM) and autoinhibitory (CaM binding) peptide in CaMKII ( e , PDB ID: 1CDM). CaM N-lobe and C-lobe are coloured yellow and green, respectively, and the orientation of IQ motifs or autoinhibitory peptide is indicated with a colour gradient (N terminus blue and C terminus red). The positions of IQ(M) amino-acid residues on the IQ domains or the 302 AI 303 amino-acid residues in the CaMKII autoinhibitory peptide are demarcated with two black lines. The cartoon figures are shown below each structure to illustrate the difference of the CaM–Na V 1.2 interactions. CaM wraps around the Na V IQ domains in the left-handed manner in contrast to the right-handed wrapping seen in Ca V structures and in CaMKII. Full size image Together with this novel interaction mode between CaM and the Na V 1.2 CTDs, our structural, biochemical and functional data provide a new framework for understanding how CaM affects Na V channels in physiology and disease. Molecular biology The following plasmids, for protein expression and purification, have been previously described: for crystallization the human Na V 1.5 CTD (amino acids 1,773–1,940) and Na V 1.2 (amino acids 1,777–1,937) were cloned into pET28 (Novagen) [21] ; the human FGF13U (accession no. NM_033642) and FGF12B were cloned into the second multiple cloning site of pETDuet-1 (Novagen) [59] ; and CaM was cloned into pSGC02 (ref. 21 ). For isothermal titration calorimetry, human Na V 1.5 CTD amino acids 1,773–1,924, Na V 1.5 CTD amino acids 1,773–1,940 (and the Ala1924Thr mutant) were cloned into pET28. For electrophysiology, Na V 1.2 was in pcDNA3.1 and FGF14b has previously been described [60] . Site-directed mutagenesis was performed with QuikChange (Stratagene). Recombinant protein expression and co-purification The three plasmids for His6-Nav1.5 CTD, FGF12B and CaM or His6-Nav1.2 CTD, FGF13U and CaM were co-electroporated into BL-21 (DE3) cells. Proteins were grown in LB medium or M9 medium as described [30] . Cells were harvested and resuspended in 300 mM NaCl, 20 mM Tris-HCl, 5 mM imidazole, 2 mM CaCl 2 , pH 7.5, supplemented with EDTA-free protease inhibitor mixture (Roche). The initial purification protocol has been previously described [30] . Additional purification was performed using gel filtration on a Superdex 200 10/300 l column on an AKTA FPLC (GE Healthcare) in 300 mM NaCl, 20 mM Tris–HCl, 5 mM imidazole, with 2 mM CaCl 2, pH 7.5. Protein concentrations were determined using UV absorbance with Thermo NANODROP and were concentrated to A 280 =12 in above buffer for crystallization. For ITC experiments, the single plasmid was electroporated into BL-21 (DE3) cells and the proteins were expressed after induction with 1 mM isopropyl-1-thio-β- D -galactopyranoside for 16 h at 20 °C. CaM protein was purified as previously described [41] . Crystallization and structure determination Crystals were grown by vapour diffusion with the sitting-drop method. His6-Nav1.5 CTD, FGF12B and Ca 2+ /CaM crystals were obtained with 20% PEG3350, 0.18 M MgSO 4 , 0.1 M sodium iodide and 2 mM CaCl 2 . His6-Nav1.2 CTD, FGF13U and CaM SeMet incorporated protein crystals were obtained with 14% pEG3350, 300 mM sodium acetate, 50 mM Tris pH 7.5 and 2 mM CaCl 2 . Before flash-freezing in liquid nitrogen, the crystals were cryoprotected by gradually increasing the concentration of glycerol in the well solution to 20%. Crystals of SeMet-substituted Na V 1.2 in complex with Ca 2+ /CaM and FGF13 diffract to 3.02 Å Bragg spacings with the space group C2 and crystals of human Na V 1.5 CTD in complex with Ca 2+ /CaM and FGF12B diffract to 3.8 Å/5.4 Å/6 Å with the space group P3 1 21 ( Table 1 ). As for the structure determination of the complex of Na V 1.2 CTD, Ca 2+ -CaM and FGF13U, experimental phases were obtained from the SeMet-substituted complex using single anomalous dispersion. After initial automatic model building, model building was completed manually. The final model contains two complexes in the asymmetric unit and is refined to R / R free of 21.5/24.6% with good geometry ( Table 1 ). The model contains residues 1,788–1,929 of Nav1.2. As for the structure determination of the complex of Na V 1.5, Ca 2+ -CaM, and FGF12B, molecular replacement was performed to obtain the phases. In brief, the EF hand domain (residue 1,786–1,896) together with FGF13 from the previous Nav1.5 CTD structure in complex with FGF13U structure and Mg 2+ -CaM (PDB ID:4DCK), IQ domain (residue 1,899–1,919) from the same complex structure, and the C-lobe of Mg 2+ -CaM (residue 85–145) were used as independent search models and used to find the solutions using Phaser [61] . After the solution was found, the N-lobe of CaM was manually placed using F o –F c map. Low-resolution structure refinement was performed using the reference model as the complex of Nav1.2, Ca 2+ /CaM and FGF13. The serious anisotropy of amplitudes were corrected using the UCLA Diffraction Anisotropy Server ( http://services.mbi.ucla.edu/anisoscale ) [62] and was used for the refinement. The final model contains one complex in the asymmetric unit and is of good quality with R / R free of 26.0/31.8% ( Table 1 ). Isothermal titration calorimetry Experiments were performed with an ITC-200 (MicroCal) at 20 °C. The solutions containing the wild-type Na V 1.5 CTD, Na V 1.2 CTD, Na V 1.2 CTD R1902C mutation, Na V 1.5 CTD amino acids 1,773–1,924, truncation mutant or A1924T mutant (25–35 μM) were titrated with one injection of 5 μl and 27 injections of 10 μl of solutions containing CaM or CaM 34 (240–310 μM). ITC experiments were repeated with different preparations and different concentrations at least three times to confirm thermodynamic parameters and stoichiometry values. The binding isotherms were analysed with a single site-binding model using the Microcal Origin version 7.0 software package (Originlab Corporation), yielding binding enthalpy (Δ H ), stoichiometry ( n ), entropy (Δ S ) and association constant ( K a ). Results are presented as mean±s.e. ; statistical significance was assessed using a two-tailed Student’s t -test and was set at P <0.05. Electrophysiology Human embryonic kidney (HEK) 293 T cells (ATCC) were cultured in DMEM supplemented with 10% heat-inactivated fetal bovine serum. The cells were plated on 60-mm tissue culture dishes and grown to 65–75% confluence, and then transfected using Lipofectamine 2000 (Invitrogen) with a total 6 μg of cDNAs encoding Na V 1.2, FGF14b, β1 and β2 at a ratio of 2:1:1. One day after transfection, the cells were re-plated on coverslips coated with 50 μg ml −1 poly-D-lysine (Sigma) for electrophysiological recordings. Transfected cells were identified by green fluorescent protein fluorescence. Na + currents were recorded using the whole-cell patch-clamp technique at room temperature (20–22 °C) 48–72 h after transfection. Electrode resistance ranged from 2.5 to 2.5 MΩ. Currents were filtered at 2.9 kHz and digitized at 20 Hz using an EPC 10 USB patch amplifier (HEKA Elektronik). Cells were allowed to stabilize for 7–10 min after the whole-cell configuration was established. Cells expressing peak current amplitude >6,000 pA were excluded from kinetic analyses because of suboptimal voltage control, as were cells exhibiting peak current amplitudes <600 pA to avoid contamination by endogenous currents. All cells were included in analyses of current density. The liquid junction potential, series resistance and leak current for these recordings were not corrected, and cells were discarded if series resistance was >8 MΩ. The bath solution contained (in mM): NaCl 124, TEA-Cl 20, CaCl 2 2.0, MgCl 2 1, HEPES 5, glucose 10, pH 7.3 (adjusted with NaOH). The intracellular ‘0 Ca 2+ ’ solution contained (in mM): CsCl 2 60, L -aspartic acid 80, 1,2-bis(o-amino phenoxy)ethane-N,N,N′,N′-tetraacetic acid (BAPTA) 10, HEPES 10, pH 7.35 (adjusted with CsOH). The intracellular ‘10 μM Ca 2+ ’ solution contained (in mM): CsCl 2 60, L-aspartic acid 80, BAPTA 1, CaCl 2 1, HEPES 10, pH 7.30 (adjusted with CsOH). Osmolarity was adjusted to 310 mOsm with sucrose for all solutions. The voltage-clamp protocols were generated using PatchMaster. Cells were voltage-clamped at a holding potential ( V h ) of −120 mV, and currents were elicited by depolarizing pulses of 40 ms from −120 to +45 mV in 5 mV increments. Current density was calculated by normalizing to cell capacitance. Activation curves were obtained by transforming current data to conductance ( G ), which was calculated from the equation G Na = I /( V − E rev ), where: I is the peak Na + current elicited by the depolarizing test potential; V is the test potential; and E rev is the calculated Na + reversal potential. The ratio G / G max was plotted against the membrane potential and fitted with the Boltzmann equation of the form: G / G max =(1+exp[( V−V 1/2 )/ k ]) −1 , where G max is the extrapolated maximum conductance, V is the test voltage, V 1/2 is the half-activation voltage and k is the slope factor. Standard two-pulse protocols were used to generate the steady-state inactivation curves: from a holding potential of −120 mV, cells were stepped to 500-ms preconditioning potentials varying between −130 and −10 mV (prepulse) in 5 mV increments, followed by a 20-ms test pulse to −20 mV. Currents ( I ) were normalized to I max and fit to a Boltzmann function of the form I / I max=1/(1+exp(( V m −/ V 1/2 )/k)) in which V 1/2 is the voltage at which half of Na V 1.5 channels are inactivated, k is the slope factor and V m is the membrane potential. Data analysis was performed using FitMaster (HEKA Elektronik) and the Origin 8 software. Results are presented as means±s.e; the statistical significance of differences between groups was assessed using a two-tailed Student’s t -test and was set at P <0.05. Accession Numbers: Atomic coordinates and structure factors for the reported crystal structures have been deposited in the Protein Data Bank under accession codes 4JPZ and 4JQ0 , for the Na V 1.2/Ca 2+ and Na V 1.5/Ca 2+ structures, respectively. How to cite this article : Wang, C. et al . Structural analyses of Ca 2+ /CaM interaction with Na V channel C termini reveal mechanisms of calcium-dependent regulation. Nat. Commun. 5:4896 doi: 10.1038/ncomms5896 (2014). Disclaimer The funders had no role in study design, data collection and analysis, decision to publish or preparation of the manuscript.